Energy transfer pathways in semiconducting carbon nanotubes revealed using two-dimensional white-light spectroscopy Thin film networks of highly purified semiconducting carbon nanotubes (CNTs) are being explored for energy harvesting and optoelectronic devices because of their exceptional transport and optical properties. The nanotubes in these films are in close contact, which permits energy to flow through the films, although the pathways and mechanisms for energy transfer are largely unknown. Here we use a broadband continuum to collect femtosecond two-dimensional white-light spectra. The continuum spans 500 to 1,300 nm, resolving energy transfer between all combinations of bandgap ( S 1 ) and higher ( S 2 ) transitions. We observe ultrafast energy redistribution on the S 2 states, non-Förster energy transfer on the S 1 states and anti-correlated energy levels. The two-dimensional spectra reveal competing pathways for energy transfer, with S 2 excitons taking routes depending on the bandgap separation, whereas S 1 excitons relax independent of the bandgap. These observations provide a basis for understanding and ultimately controlling the photophysics of energy flow in CNT-based devices. The performance of electronics, optoelectronics and energy harvesting devices is intimately related to the flow of energy and charge through their respective materials. For example, in nanostructured organic and polymer heterojunction solar cells, excitons photogenerated from solar photons must migrate through a complex energy landscape to the heterointerface where they yield charges that drive electricity [1] . The excitons’ pathway is determined by the electronic structure of the photovoltaic materials, the site-to-site energetic disorder and the inter-site coupling [2] . Direct and efficient pathways are needed so that excitons can reach the heterointerface before being trapped or annihilated by non-radiative loss mechanisms. Understanding the rates, pathways and bottlenecks is critical to controlling this energy flow and ultimately making better devices. Semiconducting carbon nanotubes (CNTs) are one candidate for next-generation semiconductor electronics [3] , near-infrared optoelectronics [4] and light absorbers or transparent conductors for solar cells [5] . Semiconducting CNTs, with controlled bandgap, can now be purified from their metallic counterparts and fabricated into mesoscale networks of densely interwoven bundles [6] , [7] . These films can be used in photovoltaics and photodetectors, in which the semiconducting tubes are photoabsorbers, analogous to electron donor polymers in polymer solar cells [8] . Like polymers, CNTs have large and tunable optical absorption and are solution processable, but nanotubes exhibit ultrafast charge and energy transport over longer distances and are more air stable [5] . While the photophysics of individual nanotubes is an established topic of study [9] , [10] , the properties of these new mesoscale films are largely unknown. In addition, the ability to control the bandgap composition of the films makes them a model system for studying exciton and charge transfer. From time-resolved photoluminescence and transient absorption spectroscopy, we know that energy transfers between nanotubes in these films and that excitons can dissociate into free carriers [11] , [12] , [13] , [14] , [15] . But the energetic manifold of these coupled thin films is extremely complex, with multiple discrete transitions per nanotube structure and multiple structures of nanotubes per film, resulting in dozens of potential relaxation pathways that are enormously difficult to resolve. Shown in Fig. 1a is the absorption spectrum for the CNT film that is the focus of this paper and has been used in previously reported prototype photovoltaic devices [5] , [16] . It is composed primarily of four different diameter nanotubes, referred to by their ( n , m ) chiral indices ( 7,5 ), ( 7,6 ), ( 8,6 ) and ( 8,7 ). Compared with the absorption spectrum of these nanotubes in solution, the bands are broadened and slightly shifted (<5 nm) [5] , [15] , indicating that the nanotube bandgap and photophysics are perturbed when the nanotubes are in close contact. A standard technique to study photophysics of CNTs and other materials is photoluminescence excitation (PLE) spectroscopy, and the PLE spectra of this film, which is shown in Fig. 1b , is similar to those previously reported for other films [5] , [17] . Each diameter tube exhibits an S 1 transition in the near-infrared (corresponding to the optical bandgap) and an S 2 transition in the visible. Only two S 2 transitions are observed because the ( 7,5 )/( 7,6 ) and ( 8,6 )/( 8,7 ) transitions overlap. The PLE measurements are performed by scanning an excitation source across the S 2 energy levels while measuring photoluminescence from the S 1 states. The resulting two-dimensional (2D) correlation map reveals the probability for exciton transfer from larger to smaller bandgap nanotubes. However, since there is no time resolution, one cannot distinguish different pathways that lead to the same emission. For example, energy transfer caused by sequential hops from larger to progressively smaller bandgap tubes could produce the same feature in a PLE spectrum as a single ‘super-hop’ directly to the lowest bandgap tube. Moreover, since energy transfer within the S 2 and the S 1 manifold of states is not measured with PLE spectroscopy, only a fraction of the possible transitions are probed, making it unclear how energy flows from S 2 to S 1 . Characterizing the pathways available for energy flow is critical for designing functional materials. 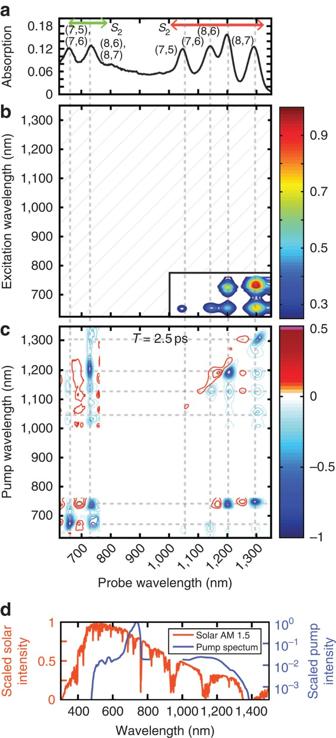Figure 1: Spectra of carbon nanotube thin films and white-light laser source. (a) Absorption spectrum, (b) PLE spectrum, (c) 2D white light spectra at pump–probe delayT=2,500 fs, and (d) log scale pump spectrum compared with the solar spectrum. The sample is composed primarily of four chiralities of nanotubes, each having anS1andS2transition labelled by their chiral index (n,m) ina. The PLE spectrum is collected as typically done by only pumping theS2transition and watching photoluminescence from theS1state. Therefore, PLE only measures cross peaks in theS2/S1quadrant. The 2D-WL spectra exhibits cross peaks in all four quadrants. Below the diagonal of the spectrum, the cross peaks are caused by energy transfer. Above the diagonal, the electronic structure intrinsic to the individual nanotubes produces the cross peaks. The intensity of each quadrant is normalized for the sake of visualization. The following figures expand on the features and dynamics measured in each of the individual quadrants. We spectrally filter out the 800 nm bandwidth from our pump, leading to the gap in the spectrum. Figure 1: Spectra of carbon nanotube thin films and white-light laser source. ( a ) Absorption spectrum, ( b ) PLE spectrum, ( c ) 2D white light spectra at pump–probe delay T =2,500 fs, and ( d ) log scale pump spectrum compared with the solar spectrum. The sample is composed primarily of four chiralities of nanotubes, each having an S 1 and S 2 transition labelled by their chiral index ( n , m ) in a . The PLE spectrum is collected as typically done by only pumping the S 2 transition and watching photoluminescence from the S 1 state. Therefore, PLE only measures cross peaks in the S 2 / S 1 quadrant. The 2D-WL spectra exhibits cross peaks in all four quadrants. Below the diagonal of the spectrum, the cross peaks are caused by energy transfer. Above the diagonal, the electronic structure intrinsic to the individual nanotubes produces the cross peaks. The intensity of each quadrant is normalized for the sake of visualization. The following figures expand on the features and dynamics measured in each of the individual quadrants. We spectrally filter out the 800 nm bandwidth from our pump, leading to the gap in the spectrum. Full size image In this article, we utilize 2D white-light spectroscopy (2D-WL) to study the exciton dynamics in thin films of CNTs. 2D-WL spectroscopy produces a correlation map analogous to PLE spectra, but since it uses a variant of transient absorption spectroscopy it has femtosecond time resolution [18] . We report a version of 2D-WL spectroscopy using a supercontinuum that spans the entire wavelength range of relevance, from 500 to 1,300 nm, and so monitors both the S 1 and S 2 states (see Fig. 1d ). The combination of ultrafast time resolution and broad bandwidth enables the kinetics for all possible pathways between all combinations of bright S 1 and S 2 states to be measured. As a result, we obtain a unified mechanism of energy transfer through these materials and observe new photophysics. 2D white-light spectroscopy Shown in Fig. 1c is a representative 2D-WL spectrum of the same film as measured with PLE spectroscopy ( Fig. 1b ), but unlike the PLE spectrum the 2D-WL spectrum exhibits peaks in all four quadrants and is time resolved (this spectrum is collected with a 2,500 fs time delay). Each of the transitions in the absorption spectrum creates a pair of diagonal peaks in the 2D-WL spectrum. The negative peak exactly on the diagonal (blue) corresponds to photobleaching of the direct bandgap transition, while the blue-shifted positive peak along the probe axis is from an excited state absorption (red) [12] , [19] . In addition to the diagonal peaks, cross peaks appear that correlate different chirality tubes. The 2D-WL spectra are plotted with the probe wavelength along the x -axis and the pump wavelengths along the y -axis so that cross peaks on the lower half of the diagonal correspond to downhill energy transfer. A cut through a specific pump wavelength (along the x -axis) is analogous to the transient absorption spectrum at that wavelength, so that the 2D-WL spectrum can be envisioned as the compilation of a continuous series of transient absorption spectra. However, as explained in the Methods section below, a Fourier transform method is used to measure the pump axis so that all pump frequencies are measured simultaneously and continuously. A continuous frequency axis avoids the one-frequency-at-a-time method of transient absorption that often leads to a piecemeal mapping of the pathways. Moreover, the 2D lineshapes resolve frequency shifts from lineshape changes, which can be difficult to discern in pump–probe spectroscopy. In essence, the 2D-WL spectra provide an instantaneous snapshot of the energy distribution in the photoexcited film. 2D-WL quadrants Each of the peaks in the 2D-WL spectrum corresponds to a specific combination of pumped and probed states. The combination of energy levels creating each observed peak is given in Supplementary Fig. 8 . To simplify the discussion, the PLE and 2D-WL spectra are sectioned into four quadrants corresponding to different combinations of pumping and probing the S 1 and S 2 states. In Fig. 2 , we present the 2D-WL spectra for the S 1 / S 1 quadrant, that is, we are pumping and probing the S 1 nanotube transition with pump–probe delays of T =100, 1,000, and 2,500 fs. These time points were chosen to illustrate the growth of new features. The blue contours correspond to photobleaching, while red contours correspond to photoabsorption. Because there is a residual amount of chirp in our laser pulses (see Supplementary Fig. 3 and Methods ), the earliest time point we plot is T =100 fs, which we define as our time resolution. A simplified energy diagram is shown to illustrate the pathway that creates each photobleaching peak. Photoabsorption pathways are not marked, but each cross peak has both a photobleach and a corresponding photoabsorption. Cross peaks to phonon side bands are also observed ( Supplementary Fig. 8 ). We plot the kinetics for each of the photobleaching cross peaks (solid lines). To quantify the timescales, the cross peak kinetics are self-consistently fit to a sum of rising and decaying exponentials ( Supplementary Methods and Supplementary Table 1 ) [11] . Figures 3 and 4 present 2D-WL spectra for the remaining three quadrants. As in the S 1 / S 1 quadrant, diagonal peaks and cross peaks are observed. Each is assigned to a specific pathway ( Supplementary Fig. 8 ). The 2D lineshapes and kinetics differ in all four quadrants, indicating that energy transfer depends on excitation state. We interpret the salient features below. 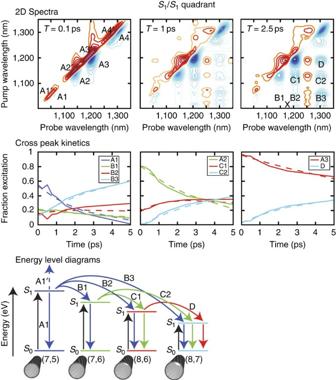Figure 2: 2D-WL spectra, kinetics, and energy levels for theS1/S1quadrant. ((a) 2D Spectra) 2D-WL spectra for pump–probe delaysT=100, 1,000 and 2,500 fs. Spectra are normalized to peak A3. The cross peaks are round and grow simultaneously, indicating energy transfer is uncorrelated and independent of bandgap. ((b) Cross peak kinetics) Kinetics of cross peaks used to obtain rates of energy transfer. Kinetics are plotted as fraction of measured photoexcitation to remove lifetime effects. Dashed lines correspond to single exponential fits to data, whose time constants are given inSupplementary Table 1and are all equal to 1 ps within error. ((c) Energy level diagrams) Energy level diagram showing the energy transfer pathway for each peak in the 2D-WL spectra used to measure the kinetics. Black arrows correspond to pumped transitions. Blue, green, and red arrows correspond to excitons that were initially excited on (7,5), (7,6) and (8,6) nanotubes, respectively. Dashed arrows correspond to excited state absorption, solid arrows correspond to ground state bleaches/stimulated emission and curved arrows correspond to energy transfer. More complete energy level diagrams are given inSupplementary Fig. 6for all of the peaks seen in the 2D-WL spectrum. Figure 2: 2D-WL spectra, kinetics, and energy levels for the S 1 / S 1 quadrant. (( a ) 2D Spectra) 2D-WL spectra for pump–probe delays T= 100, 1,000 and 2,500 fs. Spectra are normalized to peak A3. The cross peaks are round and grow simultaneously, indicating energy transfer is uncorrelated and independent of bandgap. ((b) Cross peak kinetics) Kinetics of cross peaks used to obtain rates of energy transfer. Kinetics are plotted as fraction of measured photoexcitation to remove lifetime effects. Dashed lines correspond to single exponential fits to data, whose time constants are given in Supplementary Table 1 and are all equal to 1 ps within error. (( c ) Energy level diagrams) Energy level diagram showing the energy transfer pathway for each peak in the 2D-WL spectra used to measure the kinetics. Black arrows correspond to pumped transitions. Blue, green, and red arrows correspond to excitons that were initially excited on ( 7 , 5 ), ( 7 , 6 ) and ( 8 , 6 ) nanotubes, respectively. Dashed arrows correspond to excited state absorption, solid arrows correspond to ground state bleaches/stimulated emission and curved arrows correspond to energy transfer. More complete energy level diagrams are given in Supplementary Fig. 6 for all of the peaks seen in the 2D-WL spectrum. 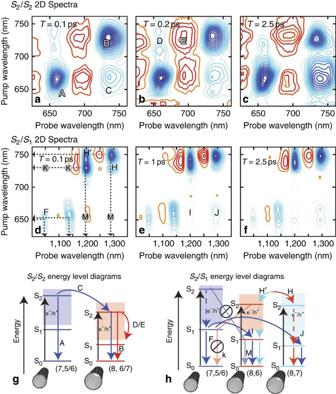Figure 3: 2D-WL spectra and energy levels for theS2/S2andS2/S1quadrants. 2D-WL spectra of theS2/S2quadrant for pump-probe delays (a)T=100fs, (b)T=200fs and (c)T=2,500 fs, normalized to peak A. Cross peaks indicate that energy transfers between nanotubes on theirS2states. The cross peaks appear at much earlier time delays than in theS1/S1quadrant, indicating much faster energy transfer. Normalized 2D-WL spectra of theS2/S1quadrant for (d)T=100fs, (e)T=1,000fs and (f)T=2,500 fs. This quadrant resolves energy transfer between the degenerateS2states. Cross peaks H and H′ indicate that energy transfers both from (8,7) to (8,6) as well from (8,6) to (8,7), which is not observed in theS1states. ((g) and (h) Energy level diagrams) Schematic energy levels and energy transfer pathways labelled by their corresponding peaks in the 2D-WL spectra. Blue, red and cyan arrows correspond to excitons that have been initially excited on the (7,5/6), (8,6) and (8,7) nanotubes, respectively. Dashed arrows correspond to relaxation between energy manifolds and curved arrows correspond to energy transfer. Cross peaks K and M are where we would expect to see signal if excitons hop directly from theS2state of one nanotube to theS1state of another. Full size image Figure 3: 2D-WL spectra and energy levels for the S 2 / S 2 and S 2 / S 1 quadrants. 2D-WL spectra of the S 2 / S 2 quadrant for pump-probe delays ( a ) T =100fs, ( b ) T =200fs and ( c ) T =2,500 fs, normalized to peak A. Cross peaks indicate that energy transfers between nanotubes on their S 2 states. The cross peaks appear at much earlier time delays than in the S 1 / S 1 quadrant, indicating much faster energy transfer. Normalized 2D-WL spectra of the S 2 / S 1 quadrant for ( d ) T =100fs, ( e ) T =1,000fs and ( f ) T =2,500 fs. This quadrant resolves energy transfer between the degenerate S 2 states. Cross peaks H and H′ indicate that energy transfers both from ( 8 , 7 ) to ( 8 , 6 ) as well from ( 8 , 6 ) to ( 8 , 7 ), which is not observed in the S 1 states. (( g ) and ( h ) Energy level diagrams) Schematic energy levels and energy transfer pathways labelled by their corresponding peaks in the 2D-WL spectra. Blue, red and cyan arrows correspond to excitons that have been initially excited on the ( 7 , 5 / 6 ), ( 8 , 6 ) and ( 8 , 7 ) nanotubes, respectively. Dashed arrows correspond to relaxation between energy manifolds and curved arrows correspond to energy transfer. Cross peaks K and M are where we would expect to see signal if excitons hop directly from the S 2 state of one nanotube to the S 1 state of another. 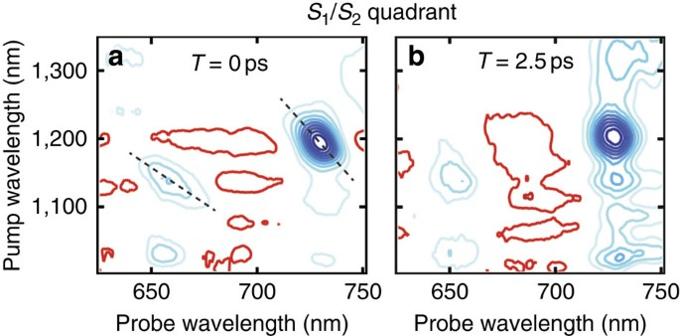Figure 4: 2D-WL spectra of theS1/S2quadrant. 2D-WL spectra of theS1/S2quadrant for (a)T=0and (b) 2,500 fs. These cross peaks are not caused by energy transfer, but result from a change in theS2electronic state by pumping theS1state. The cross peaks are elongated anti-diagonally, indicating an anticorrelation in the frequency distribution of theS1andS2states. Dashed lines are guides to the eye to highlight the anti-correlated lineshapes of the cross peaks. Full size image Figure 4: 2D-WL spectra of the S 1 / S 2 quadrant. 2D-WL spectra of the S 1 / S 2 quadrant for ( a ) T=0 and ( b ) 2,500 fs. These cross peaks are not caused by energy transfer, but result from a change in the S 2 electronic state by pumping the S 1 state. The cross peaks are elongated anti-diagonally, indicating an anticorrelation in the frequency distribution of the S 1 and S 2 states. Dashed lines are guides to the eye to highlight the anti-correlated lineshapes of the cross peaks. Full size image Photoexcitation transfer between bandgap S 1 states Each quadrant of the 2D-WL spectra probes photoexcitation transfer among a different class of electronic states. Photoexcitation of S 1 lies below the ionization threshold and so excitons, but not charges, are generated [20] . All of the cross peaks in this quadrant appear on the lower half of the diagonal, indicating that energy transfer occurs downhill from larger to smaller bandgap tubes. These cross peaks are not seen in the solution samples of uncoupled nanotubes ( Supplementary Fig. 5 ), confirming that they arise from energy transfer. Except for cross peaks to phonon modes (peak X, which grow in after ∼ 300 fs and then decay similar to the diagonal peaks), the cross peaks grow in simultaneously, indicating that exciton transfer is equally likely between any downhill combination of nanotubes. Moreover, the cross peaks are round, whereas the diagonal peaks are elongated. The 2D lineshapes of cross peaks measure joint frequency correlations and will appear elongated for correlated frequency distributions [21] . Round cross peaks signify uncorrelated energy transfer, that is, an exciton generated anywhere within the distribution of energies of a particular bandgap nanotube has equal probability of transferring to another nanotube anywhere within the acceptor’s distribution of energies. Thus, the inhomogeneity of the bandgap transitions does not impact energy transfer. We quantify these observations by fitting with a simple model using single exponentials ( Fig. 2 ), all of which have time constants between 1 and 3 ps. Taking into account the fitting error, the time constants are indistinguishable. Thus, it is equally likely for an S 1 exciton to relax to the next smallest bandgap as it is to ‘super-hop’ directly to the smallest bandgap tube. Non-exponential dynamics would be observed if hopping were sequential from large to small bandgap, or presumably if multi-exciton effects were present [22] . Based on the quality that the data can be fit with single exponentials, the similarity of the transfer rates and a lack of correlation, we conclude that transfer is independent of the spectral overlap, ruling out Förster resonance energy transfer between bright states as the rate limiting mechanism. One possibility is that inter-nanotube energy transfer proceeds through Dexter, exciton tunnelling or another non-Förster mechanism [23] , [24] . Another possibility is that inter-nanotube transfer rates are diffusion limited as in previous transient absorption experiments, pumping the S 2 states and probing the S 1 states led to the conclusions that there are ‘hot spots’ for energy transfer to occur between nanotubes, such as at fibre–fibre intersections, and that diffusion to these ‘hot spots’ can limit kinetics [25] . These findings are interesting because previous reports concluded that energy transfer between nanotubes was dominated by a Förster resonance energy transfer process [13] , [26] , as one might expect for molecules with such large transition dipoles, whereas we find that energy transfer between nanotubes is limited by a non-resonant process. Photoexcitation transfer between S 2 states Photoexcitation transfer also occurs between S 2 states, as revealed by cross peaks appearing within 100 fs in the S 2 / S 2 quadrant ( Fig. 3 , peak C), but the pathways for visible excitation are more complex. Prior work concluded that energy transfer in the S 2 manifold does not take place because of momentum mismatch and fast relaxation to S 1 ( ∼ 40 fs) [14] . The 2D-WL spectra clearly show that transfer among S 2 states is fast enough to compete with relaxation to S 1 , enabling energy redistribution on the S 2 manifold. Thus, energy transfer on both the S 2 and S 1 states are contributing to the features observed in the PLE spectra. Due to the degeneracies, the S 2 / S 2 quadrant only resolves energy transfer between ( 7,5/6 ) to ( 8,6/7 ) tubes. However, the remaining S 2 pathways can be monitored in the S 2 / S 1 quadrant because the S 1 transitions are all well-resolved ( Fig. 3 ). Based on the frequencies of the peaks (dashed lines), the S 2 transitions of the ( 7,5 ) and ( 7,6 ) tubes are at 654 nm and 656 nm, respectively, while the ( 8,6 ) and ( 8,7 ) tubes are at 731 nm and 750 nm, respectively. Interestingly, cross peaks are observed both above and below the diagonal of this quadrant, as marked by cross peaks H and H′. H and H′ indicate energy transfer from ( 8,6 ) to ( 8,7 ) as well as from ( 8,7 ) to ( 8,6 ), in contrast to S 1 energy transfer in which only the former process occurs. From these features we conclude that the near degeneracy of the S 2 states of the ( 8,6 ) and ( 8,7 ) tubes enables energy transfer to occur in either direction. Moreover, energy transfer between these nearly degenerate states is extremely fast, because unlike any other peaks in the 2D-WL spectra (other than the phonon side bands), peaks H and H′ are already very intense at T = 100 and do not appreciably grow in intensity with time delay. Thus, 100 fs is an upper bound for transfer between S 2 states. Other pathways that might contribute to these peaks are eliminated by examining other quadrants, for example, these peaks could be generated by S 2 relaxation to S 1 followed by inter-nanotube transfer among S 1 states, but this pathway is ruled out because the S 1 / S 1 quadrant cross peaks appear in picoseconds not femtoseconds. An interesting consequence of the S 2 dynamics is that visible S 2 excitation of an ( 8 , 7 ) tube can transfer to an ( 8 , 6 ) tube before relaxing to S 1 , resulting in a pathway that deposits more energy on the S 1 state of the ( 8 , 6 ) tube than if the ( 8 , 7 ) S 1 bandgap transition was irradiated directly. Similar conclusions are drawn for transitions between the ( 7 , 5 ) and ( 7 , 6 ) tubes, although the cross peaks are not as well-resolved (appearing as shoulders) because these transitions are more closely spaced. Not all downhill pathways are observed. We see no evidence for relaxing directly from the S 2 state of one nanotube to the S 1 state of another, which is energetically downhill (grey transitions in Fig. 3 , peaks K and M). Peaks I and J cannot result from this pathway because the lifetime of the S 2 state is ∼ 40 fs [14] , but these cross peaks are not observed until ∼ 1 ps, which corresponds to the time scale for energy transfer on the S 1 manifold. Apparently, coupling between S 1 and S 2 states on different nanotubes is not large enough to activate this pathway. Thus, intertube energy transfer occurs among S 2 states and among S 1 states, but only intratube transfer connects the two manifolds. Possible signatures of charge transfer Besides exciton transfer, we also observe features that we believe are due to charge generation. In the S 2 / S 2 quadrant, weak cross peaks are observed on the upper half of the spectrum (peaks D and E). These peaks cannot be caused by uphill energy transfer because the energy difference between ( 7 , 5 / 6 ) and ( 8 , 6 / 7 ) S 2 states is ≫ kT nor can they be caused by direct relaxation from S 2 to S 1 of different bandgap tubes, which is a process ruled out in the previous paragraph. An alternative hypothesis is that peaks D and E originate from a Stark shift arising from free carrier generation. We estimate that the electric field necessary to produce this shift would be ∼ 87 V μm −1 , which is consistent with other reported electric field-induced shifts in CNTs [27] , [28] . This hypothesis is supported because peaks D and E in the S 2 / S 2 quadrant have no equivalent features in other quadrants and it is known that the S 2 excitation overlaps the free carrier continuum, whereas the S 1 states are too low in energy to generate free carriers [27] . Photogenerated free carriers on ( 8 , 6 / 7 ) nanotubes could perturb the S 2 of nearby ( 7 , 5 / 6 ) nanotubes, Stark shifting the electronic states to yield a photoabsorption and photobleach, as previously assigned using transient absorption spectroscopy [12] , [29] . The free carrier signals are much weaker than the exciton peaks, which is consistent with prior work that showed charge generation is a minority process [12] , [30] . Unlike pump–probe measurements, these 2D-WL cross peaks have no other overlapping features and so are background free, allowing the free carrier dynamics to be resolved at very early time delays. Auger ionization has also been shown to produce free carriers [31] , however based on our signal intensity, we believe that we are in a regime where most nanotubes have a single exciton initially excited (see Supplementary discussion ) [30] . Auger ionization should also yield free carriers through S 1 excitation, but this is not observed. Anti-correlated electronic states Other interesting features appear in the S 1 / S 2 quadrant ( Fig. 4 ). We observe cross peaks between S 1 and S 2 states of the same but not different chirality tubes. These cross peaks cannot be due to exciton transfer, because pumping S 1 is too low in energy to transfer to S 2 . Instead, these cross peaks are measuring the electronic correlation internal to the nanotubes. In other words, they arise because the S 1 and S 2 electronic states are not perfectly orthogonal [19] . The centre line slopes are negative and elongated perpendicular to the diagonal (the dashed line is a visual guide), which indicates that the S 1 and S 2 transitions are anti-correlated. Anticorrelation means that large S 2 transitions are correlated with small S 1 bandgaps and vice versa for a given ( n , m ) nanotube ( Supplementary Fig. 8 ) (no correlation would produce round cross peaks). For nanotubes dispersed in solution, we only observe weak anticorrelation ( Supplementary Fig. 7 ), leading us to conclude that the anticorrelation in energy levels is caused by the film casting. Stranks et al . [32] observed anti-correlated peak shifts in CNT absorption and emission spectra for nanotubes wrapped with rigid porphyrin molecules (but not for PFO wrapping as in our samples), which they attributed to localized strain of the nanotube. Alternative theories for the anti-correlated lineshape are considered in the Supplementary discussion , but it appears that strain caused by surface tension during film casting, differences in thermal expansion (our films are annealed) or mechanical stress on the nanotubes lowers the S 1 while raising the S 2 energy gap (and vice versa ). 2D lineshapes measure spectral diffusion 2D-WL spectroscopy also probes dynamics through the time evolution of the 2D lineshapes. The elongation of the diagonal peaks measures the distribution of energies that the bandgap can span for each particular ( n , m ) nanotube, that is, the inhomogeneity of the bandgap transitions [33] . Thus, the peak elongation along the diagonal is a measure of the energetic disorder in the film. In all quadrants, the peak shapes become rounder with time delay, indicating spectral diffusion. Spectral diffusion could be caused by the diffusion of excitons as they sample different environments along the tube lengths, by relaxation of the dielectric on exciton formation [33] , or by energy transfer among nanotubes of the same chirality. Measuring the kinetics of the 2D peak shapes probes the dynamics of these processes [33] . Thus, after ∼ 2 ps when the peaks are mostly round, the excitons have fully sampled the available environment. We point out that, on the larger bandgap nanotubes, the peaks are still elongated along the diagonal after 2 ps. We believe that this long-lived inhomogeneity is a signature of trapped excitons, because trapped excitons would not be able to fully sample the potential energy landscape. Experiments are underway to contrast the 2D lineshapes of coupled and uncoupled nanotubes to test this hypothesis and better understand the effects of nanotube couplings. Using 2D-WL spectroscopy, we have resolved all possible pathways for energy transfer that can be optically probed in this CNT thin film. The bird’s-eye view of a 2D-WL spectrum provides an unprecedented level of clarity because of the continuous and broad wavelength range combined with femtosecond time resolution. In many instances, unambiguous peak assignments required self-consistent checks between multiple quadrants, which are not often reported with standard transient absorption spectroscopy. We found that all pathways are equally likely on the S 1 manifold, indicating that Förster energy transfer is not the rate limiting step for exciton transfer. Energy transfer on the S 2 manifold is 10 times faster and can transfer on sub-100 fs timescales between degenerate tubes. As a result, redistribution between S 2 states competes with relaxation to the S 1 states, producing more complex pathways for excitons created from visible than infrared light. These principles will be useful for guiding the design of mesoscale thin films of semiconducting CNTs used in photovoltaics and other optoelectronics. Sample preparation The procedure used to prepare semiconducting CNTs is adopted from Nish et al . [6] and is described in more detail in the Supplementary Methods . It uses poly(9,9-dioctylfluorenyl-2,7-diyl) (PFO, American Dye Source) mixed with high pressure carbon monoxide (HiPco) single-wall CNT mud (NanoIntegris) (5.3% carbon by weight) to selectively purify the semiconducting nanotubes from the metallic tubes and impurities using ultracentrifugation. Once purified, excess PFO is removed, resulting in a CNT:PFO solution with a weight ratio of 1:2 that is used to drop cast a film on a 1 in × 1 in substrate of indium tin oxide on glass. The resulting CNT film is annealed at 150 °C for 30 min under N 2 atmosphere to remove any residual solvent and encapsulated with an epoxied cover slip to exclude oxygen. Prior to 2D-WL measurements, photoluminescence emission spectra (Horiba Scientific NanoLog FluoroLog3) are collected to confirm that energy transfer is observed within the films ( Fig. 1b and Supplementary Fig. 1 ). 2D-WL spectrometer There are many different spectrometer designs for collecting 2D spectra [18] , [34] , [35] , [36] , [37] , [38] , [39] , [40] , [41] , [42] . Our spectrometer design, shown in Supplementary Fig. 2 and described more fully in the Supplementary Methods , is very similar to a transient absorption spectrometer. The main difference is that the pump pulse has been shaped into a pair of collinear pulses using birefringent wedges [43] . Alternatively, one can use an interferometer [37] , [44] or pulse shaper [45] , [46] to create the pulse pairs. To generate the white-light continuum, <1 μJ from the output of a Ti:Sapphire regenerative amplifier (800 nm, 150 fs, 1 kHz) is focused into each of two YAG crystals that are 4-mm thick [47] . A representative pump spectrum is shown in Fig. 1d and compared with the solar spectrum. To limit pulse broadening, the optical path for the white light of the probe only uses reflective optics. For the pump beam, the white light must pass through the birefringent wedges, and so we compensate for pump dispersion using a prism compressor. Because of the large bandwidth of our optical pulses ( ∼ 250 THz), the wedges introduce a significant dispersion to our pulses and so prisms cannot compress the entire bandwidth at once. As a result, the 2D-WL spectra are collected in two halves, with the pump pulses either compressed for the S 1 or the S 2 transition. Optical Kerr effect cross-correlations using the 800 nm laser pulses in CaF 2 are used to measure the group delay of the pump and probe pulses ( Supplementary Fig. 3 ), which sets our time resolution to <150 fs for either wavelength range. We also use the prism compressor to filter out the fundamental 800 nm light, although there are no resonant transitions in these samples at 800 nm. To make sure that the pump pulse is only creating one exciton per nanotube, the white light is defocused to an intensity that only produces approximately one exciton per 400 nm, which corresponds to the average length of the CNTs. A number of control experiments are presented in the Supplementary Discussion to support this conclusion. To collect the 2D data, the time delay between the pair of pump pulses is scanned while measuring the spectrum of the probe. To generate the pump axis of the 2D spectrum, the data are Fourier transformed and phased according to the projection slice theorem [48] . The Fourier transform separates out all of the frequency components spanned by the pump bandwidth, analogous to scanning a continuous series of narrowband pump pulses such as with a NOPA. Vertical lines in the spectra are due to tails of the Lorentzian lineshapes. Horizontal tails are not as prominent because of destructive interference of the bleach and excited state absorption [21] . How to cite this article: Mehlenbacher, R. D. et al . Energy transfer pathways in semiconducting carbon nanotubes revealed using two-dimensional white-light spectroscopy. Nat. Commun . 6:6732 doi: 10.1038/ncomms7732 (2015).